Overexpression of Atg5 in mice activates autophagy and extends lifespan Autophagy has been implicated in the ageing process, but whether autophagy activation extends lifespan in mammals is unknown. Here we show that ubiquitous overexpression of Atg5, a protein essential for autophagosome formation, extends median lifespan of mice by 17.2%. We demonstrate that moderate overexpression of Atg5 in mice enhances autophagy, and that Atg5 transgenic mice showed anti-ageing phenotypes, including leanness, increased insulin sensitivity and improved motor function. Furthermore, mouse embryonic fibroblasts cultured from Atg5 transgenic mice are more tolerant to oxidative damage and cell death induced by oxidative stress, and this tolerance was reversible by treatment with an autophagy inhibitor. Our observations suggest that the leanness and lifespan extension in Atg5 transgenic mice may be the result of increased autophagic activity. Autophagy is an evolutionarily conserved process for cellular homeostasis through the degradation of long-lived proteins and functionally redundant or damaged intracellular organelles in lysosomes [1] . Autophagy provides energy through the turnover of intracellular proteins and organelles to guarantee rejuvenation and adaptation in various conditions. Autophagy also functions as the mechanism for the removal of unwanted cellular structures by the degradation of excess or injured organelles, for example, redundant peroxisomes, damaged mitochondria and endoplasmic reticulum [2] . Numerous studies have shown that autophagy has an important role in diverse physiological and pathological processes, including cell growth, cell differentiation and development, immune responses, cancer, neurodegeneration, infection and metabolic syndrome [3] , [4] , [5] . Beyond these aforementioned functions, autophagy has also been implicated in ageing, at least in model organisms. The first genetic connection between autophagy and ageing was established in Caenorhabditis elegans . The knockdown of beclin 1 in daf-2 mutants drastically reduces their lifespan [6] , [7] , [8] . In Drosophila melanogaster , inhibition of mTOR signalling extends lifespan, as it does in yeast and C. elegans [9] , [10] . On the other hand, there is no evidence in mice showing a role of autophagy in longevity because genetic inhibition of autophagy genes results in embryonic or neonatal lethality. In addition, pharmacological approaches using resveratrol [11] , spermidine [12] and rapamycin, an mTOR inhibitor and immunosuppressant [13] , provide an indication that the activation of autophagy, as well as other processes, may be associated with longevity in eukaryotes and mice [11] , [12] , [13] . However, critical evidence that autophagy contributes to longevity in mammals is not yet available. The molecular mechanism of autophagy involves several conserved autophagy-related genes ( Atg ) and these genes have multiple functions in various physiological contexts. Among these genes, Atg5 protein in a conjugated form with Atg12 and Atg8 (LC3) are involved in the early stages of autophagosome formation [14] . Especially, Atg5 is important for development, cell differentiation and maintenance of homeostasis, including early neonatal starvation [15] . Atg5-knockout mice die at the neonatal stage [15] and Atg5-deficient mice, specifically in neural cells, and mice with a mosaic deletion of Atg5 develop progressive deficits in motor function from neurodegeneration [16] and benign liver adenomas [17] , respectively. In addition, Atg5 is downregulated at the transcriptional level during ageing in humans and is also upregulated by endoplasmic reticulum (ER) stress to affect autophagy [18] , [19] . Here, to address the role of autophagy activation in mammalian longevity by genetic approaches, we generated transgenic ( Tg ) mice expressing Atg5 ubiquitously to enhance autophagy activity. We report that the median and maximal lifespan of both male and female Atg5 Tg mice are extended together with a lean phenotype, increased insulin sensitivity and resistance to oxidative stress. Atg5 Tg mice exhibit an extended lifespan To address the role of autophagy activation in mammalian longevity, we generated Tg mice expressing Atg5 ubiquitously (Atg5 Tg ). Atg5 cDNA was inserted into an expression vector ( p CAGGS) driven by the cytomegalovirus enhancer and the chicken β-actin promoter [20] . Unlike the lethal phenotype of Atg5-knockout mice after birth [15] , Atg5 Tg mice grew normally and were healthy without any detectible symptoms of age-related diseases, including skin ulcerations and atrophy, fertility ( Supplementary Table S1 ) and blood cell index ( Supplementary Table S2 ). There was also no significant difference between the ability of wild-type (WT) and Atg5 Tg mice to remember the correct arm of a Y-maze ( Supplementary Fig. S1 ). When we evaluated the longevity of Atg5 Tg mice and their WT littermates using a Kaplan–Meier survival curve, the combined data for males and females showed that the maximum lifespan of WT mice and Atg5 Tg mouse line 25 (mice no. 25) were 781±22 and 900±34 days (s.e.m., P <0.01), respectively, and the median lifespan of Atg5 Tg mice no. 25 was 119 days or ~17% longer than that of WT mice ( χ 2 =17.32, s.e.m., P <0.001) ( Fig. 1a ). Analysis of each sex separately revealed that the median lifespan of male and female Atg5 Tg mice no. 25 was similarly increased by 120 and 117 days, respectively ( Fig. 1b,c ), indicating no gender-dependent difference in the extended lifespan. Moreover, when we analysed three more lines of Atg5 Tg mice that showed similar levels of Atg5 expression with Atg5 Tg mice no. 25 ( Fig. 1g ), the median lifespan of Atg5 Tg mice no. 43 ( Fig. 1d ), no. 47 ( Fig. 1e ), and no. 471 ( Fig. 1f ) was increased by 113, 100 and 130 days, respectively. 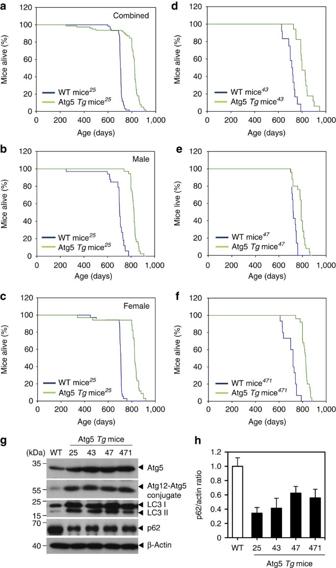Figure 1: Lifespan analysis of Atg5Tgmice. (a) Kaplan–Meier survival curves of combined male and female WT and Atg5Tgmice no. 25 (P<0.001;n=65 for WT mice andn=70 for Atg5Tgmice). (b,c) Lifespan extension in male Atg5Tgmice no. 25 (P<0.001;n=32 for WT mice andn=36 for Atg5Tgmice no. 25) (b) and female Atg5Tgmice no. 25 (P<0.001;n=33 for WT mice andn=34 for Atg5Tgmice no. 25) (c). (d–f) Kaplan–Meier survival curves of combined male and female WT and Atg5Tgmice no. 43 (d), no. 47 (e) and no. 471 (f) (P<0.001;n=25 for WT mice andn=30 for Atg5Tgmice).P-values were calculated using the log-rank test. (g) Expression levels of Atg5 and Atg12-Atg5 conjugate, the conversion of LC3 I into LC3 II, and p62 level in the hearts of Atg5Tgmice. Whole-tissue extracts were prepared from 3-month-old Atg5Tgmice and WT littermates, and analysed by western blotting using the indicated antibodies. β-Actin served as a control. (h) Densitometric analysis of the signals on the blots shown in (g). The bars represent the mean±s.d. (n=3). Figure 1: Lifespan analysis of Atg5 Tg mice. ( a ) Kaplan–Meier survival curves of combined male and female WT and Atg5 Tg mice no. 25 ( P <0.001; n =65 for WT mice and n =70 for Atg5 Tg mice). ( b , c ) Lifespan extension in male Atg5 Tg mice no. 25 ( P <0.001; n =32 for WT mice and n =36 for Atg5 Tg mice no. 25) ( b ) and female Atg5 Tg mice no. 25 ( P <0.001; n =33 for WT mice and n =34 for Atg5 Tg mice no. 25) ( c ). ( d – f ) Kaplan–Meier survival curves of combined male and female WT and Atg5 Tg mice no. 43 ( d ), no. 47 ( e ) and no. 471 ( f ) ( P <0.001; n =25 for WT mice and n =30 for Atg5 Tg mice). P -values were calculated using the log-rank test. ( g ) Expression levels of Atg5 and Atg12-Atg5 conjugate, the conversion of LC3 I into LC3 II, and p62 level in the hearts of Atg5 Tg mice. Whole-tissue extracts were prepared from 3-month-old Atg5 Tg mice and WT littermates, and analysed by western blotting using the indicated antibodies. β-Actin served as a control. ( h ) Densitometric analysis of the signals on the blots shown in ( g ). The bars represent the mean±s.d. ( n =3). Full size image Transgenic Atg5 enhances autophagy in mice We analysed the expression levels of endogenous and transgenic Atg5 in the tissues of WT and Atg5 Tg mice no. 25 using western blotting. Compared with WT mice, the expression of Atg5 was highly increased in the lung, heart, liver and muscle (≥2-fold) and marginally increased in the brain of Atg5 Tg mice ( Fig. 2a ). Accordingly, the levels of Atg12-Atg5 conjugate and LC3 I and the conversion of LC3 I to LC3 II, which are markers of autophagy [14] , were apparently higher in almost all of the tissues of Atg5 Tg mice compared with WT mice. Consistently, the levels of p62 protein, an indicator of ubiquitinated protein [21] , were drastically decreased in the tissues of Atg5 Tg mice ( Fig. 2a ). Although there were marginal differences in the expression levels of p62 and Atg5 during ageing of WT mice, autophagy activity was higher in the heart of all ages of Atg5 Tg mice than WT mice ( Supplementary Fig. S2 ). 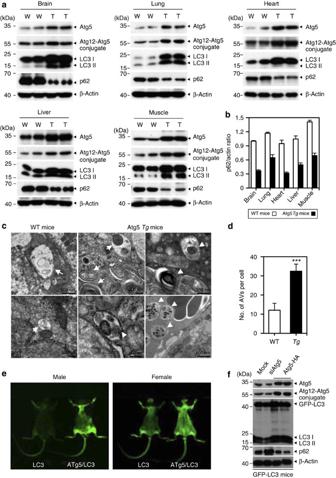Figure 2: Enhanced autophagy in Atg5Tgmice. (a) Western blot analysis showing enhanced levels of Atg5, Atg12-Atg5 conjugate and LC3 conversion, and reduced p62 levels in the indicated tissues of 18-month-old Atg5Tgmice no. 25 (T) and WT mice (W). (b) Densitometric analysis of the signals on the blots shown in (a). (c) Electron microscopy images of autophagosomes (arrows) and late-autophagic compartments (arrowheads) in the liver tissues of 18-month-old Atg5Tgmice no. 25 and WT mice. Scale bars are indicated. (d) The numbers of autophagosomes and autolysosomes per cell (n=50) in the electron microscopic images shown in (c) were counted. The bars represent the mean±s.d. ***P<0.0001 versus control; Student’st-test. (e) Fluorogenic comparison of basal autophagy activity between GFP-LC3Tgmice and Atg5/GFP-LC3 doubleTgmice. Whole bodies of 8-week-old male (left) and female (right) GFP-LC3Tg(LC3), and Atg5/GFP-LC3Tgmice (Atg5/LC3) were visualized using a Kodak Image Station 4000MM equipped with a filter set for FITC (Kodak Molecular Imaging Software, Version 4.0). (f) Western blot analysis showing autophagy markers in the liver of GFP-LC3 mice. GFP-LC3 mice were injected for 5 days with siRNA-Atg5 or Atg5-HA cDNA through the tail vein. Whole-liver tissue lysates were prepared and subjected to immunoblotting using the indicated antibodies. β-Actin served as a control. Figure 2: Enhanced autophagy in Atg5 Tg mice. ( a ) Western blot analysis showing enhanced levels of Atg5, Atg12-Atg5 conjugate and LC3 conversion, and reduced p62 levels in the indicated tissues of 18-month-old Atg5 Tg mice no. 25 (T) and WT mice (W). ( b ) Densitometric analysis of the signals on the blots shown in ( a ). ( c ) Electron microscopy images of autophagosomes (arrows) and late-autophagic compartments (arrowheads) in the liver tissues of 18-month-old Atg5 Tg mice no. 25 and WT mice. Scale bars are indicated. ( d ) The numbers of autophagosomes and autolysosomes per cell ( n =50) in the electron microscopic images shown in ( c ) were counted. The bars represent the mean±s.d. *** P <0.0001 versus control; Student’s t -test. ( e ) Fluorogenic comparison of basal autophagy activity between GFP-LC3 Tg mice and Atg5/GFP-LC3 double Tg mice. Whole bodies of 8-week-old male (left) and female (right) GFP-LC3 Tg (LC3), and Atg5/GFP-LC3 Tg mice (Atg5/LC3) were visualized using a Kodak Image Station 4000MM equipped with a filter set for FITC (Kodak Molecular Imaging Software, Version 4.0). ( f ) Western blot analysis showing autophagy markers in the liver of GFP-LC3 mice. GFP-LC3 mice were injected for 5 days with siRNA-Atg5 or Atg5-HA cDNA through the tail vein. Whole-liver tissue lysates were prepared and subjected to immunoblotting using the indicated antibodies. β-Actin served as a control. Full size image From electron microscopic analysis, we observed that the numbers of autophagosomes and late-autophagic compartments were increased by threefold in the liver of Atg5 Tg mice ( Fig. 2c,d ). Further, we crossed Atg5 Tg mice with GFP-LC3 Tg mice, a model mouse to visualize autophagosomes [22] , to obtain double Tg mice expressing both Atg5 and GFP-LC3 (Atg5/GFP-LC3 Tg ). When visualized under a Kodak FITC imaging station, male and female Atg5/GFP-LC3 double Tg mice showed enhanced fluorescence intensity of GFP-LC3 throughout their bodies, especially in the muscle, compared with GFP-LC3 Tg mice ( Fig. 2e ). When Atg5 expression was reduced in the liver of GFP-LC3 mice by tail vein injection of small interfering RNA (siRNA) against Atg5 (siRNA-Atg5), Atg12-Atg5 conjugate and LC3 conversion were reduced and p62 protein level increased ( Fig. 2f ). Conversely, enhanced expression of Atg5 by tail vein injection of Atg5 cDNA resulted in increased autophagy activity in the liver ( Fig. 2f ). Further, ectopic expression of Atg genes, including Atg5 , in mammalian cells, enhances autophagy activity ( Supplementary Fig. S3 ). Taken together, we suggest that the increased expression of Atg5 in mice enhances autophagy activity. Atg5 Tg mice are lean and show improved insulin sensitivity In addition to enhanced longevity, the body weight of aged Atg5 Tg mice was apparently reduced. Compared with WT littermates, Atg5 Tg mice showed leanness on a regular diet ( Fig. 3a ). When we monitored body weight over 24 months on a regular diet, both Atg5 Tg mice and WT littermates gained weight at a similar rate at a young age. However, after 12 months, Atg5 Tg mice weighed on average 12% less than WT mice ( Fig. 3b ). We did not detect a significant difference in food intake between WT and Atg5 Tg mice ( Fig. 3c ). Along with their reduction in total body weight, the gonadal fat pads of Atg5 Tg mice weighed much less than those of WT mice and this difference was more prominent in aged mice (18 months) ( Fig. 3d ). Compared with WT mice, the weight of the visceral and subcutaneous fat pads was also reduced in Atg5 Tg mice ( Fig. 3e,f ). Thus, transgenic expression of Atg5 in mice results in leaner mice and confers resistance to age-associated obesity. 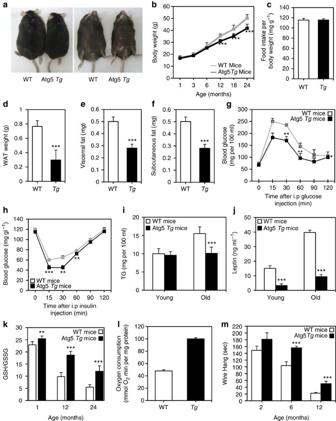Figure 3: Metabolic characteristics of lean Atg5Tgmice. (a) Representative physical pictures of 18-month-old WT and Atg5Tgmice fed with a regular diet. (b) Body weight chart of ageing-induced obesity in WT and Atg5Tgmice. The mice were fed with a regular diet for 24 months (n=180-–250) and their body weights were monitored monthly. The bars represent the mean±s.d. ***P<0.0001 versus control; Student’st-test. (c) Average daily oral food intake normalized to body weight, measured on regular diet. The food intake of mice (n=18–24) was measured for 2 weeks at 3-, 6-, 12- and 18-month-old age. (d) Quantification of gonadal fat pads from 18-month-old mice (n=11). ***P<0.0001 versus control; Student’st-test. (e,f) Quantification of visceral (e) and subcutaneous (f) fat pads of 18-month-old mice (n=6). ***P<0.0001 versus control; Student’st-test. (g) Enhanced glucose tolerance of Atg5Tgmice. WT and Atg5Tgmice were starved overnight and then given with an i.p injection of glucose (1 mg g−1body weight). The results are the mean±s.d. of 12-week-old WT and Atg5Tgmice (n=12). *P<0.01, **P<0.001, ***P<0.0001 versus control; Student’st-test. (h) Enhanced insulin sensitivity of Atg5Tgmice. WT and Atg5Tgmice were starved for 6 h and then i.p injected with 0.75 IU soluble insulin. *P<0.01, **P<0.001 versus control; Student’st-test. (i) Plasma levels of triglycerol (TG) in WT and Atg5Tgmice. The mice were fasted for 3 h before measurement. Young mice (4-week old,n=8); old mice (18-month old,n=8). ***P<0.0001 versus control; Student’st-test. (j) Plasma leptin levels in WT and Atg5Tgmice (n=8–12). ***P<0.0001 versus control; Student’st-test. (k) GSH/GSSG ratio in the liver (n=4 males, three times trial). **P<0.001, ***P<0.0001 versus control; Student’st-test. (l) Respiration rates of mitochondria in WT and Atg5TgMEFs (n=2). (m) Wire-hang endurance test of Atg5Tgand WT mice (n=10). All the bars represent the mean±s.d. ***P<0.0001 versus control; Student’st-test. Figure 3: Metabolic characteristics of lean Atg5 Tg mice. ( a ) Representative physical pictures of 18-month-old WT and Atg5 Tg mice fed with a regular diet. ( b ) Body weight chart of ageing-induced obesity in WT and Atg5 Tg mice. The mice were fed with a regular diet for 24 months ( n =180-–250) and their body weights were monitored monthly. The bars represent the mean±s.d. *** P <0.0001 versus control; Student’s t -test. ( c ) Average daily oral food intake normalized to body weight, measured on regular diet. The food intake of mice ( n =18–24) was measured for 2 weeks at 3-, 6-, 12- and 18-month-old age. ( d ) Quantification of gonadal fat pads from 18-month-old mice ( n =11). *** P <0.0001 versus control; Student’s t -test. ( e , f ) Quantification of visceral ( e ) and subcutaneous ( f ) fat pads of 18-month-old mice ( n =6). *** P <0.0001 versus control; Student’s t -test. ( g ) Enhanced glucose tolerance of Atg5 Tg mice. WT and Atg5 Tg mice were starved overnight and then given with an i.p injection of glucose (1 mg g −1 body weight). The results are the mean±s.d. of 12-week-old WT and Atg5 Tg mice ( n =12). * P <0.01, ** P <0.001, *** P <0.0001 versus control; Student’s t -test. ( h ) Enhanced insulin sensitivity of Atg5 Tg mice. WT and Atg5 Tg mice were starved for 6 h and then i.p injected with 0.75 IU soluble insulin. * P <0.01, ** P <0.001 versus control; Student’s t -test. ( i ) Plasma levels of triglycerol (TG) in WT and Atg5 Tg mice. The mice were fasted for 3 h before measurement. Young mice (4-week old, n =8); old mice (18-month old, n =8). *** P <0.0001 versus control; Student’s t -test. ( j ) Plasma leptin levels in WT and Atg5 Tg mice ( n =8–12). *** P <0.0001 versus control; Student’s t -test. ( k ) GSH/GSSG ratio in the liver ( n =4 males, three times trial). ** P <0.001, *** P <0.0001 versus control; Student’s t -test. ( l ) Respiration rates of mitochondria in WT and Atg5 Tg MEFs ( n =2). ( m ) Wire-hang endurance test of Atg5 Tg and WT mice ( n =10). All the bars represent the mean±s.d. *** P <0.0001 versus control; Student’s t -test. Full size image Because the gain or loss of body weight is usually associated with insulin sensitivity [23] , [24] , the mice were subjected to insulin- and glucose-tolerance tests (ITT and GTT). Upon glucose stimulation for the GTT, Atg5 Tg mice exhibited significantly reduced blood glucose levels ( Fig. 3g ), which may be derived from elevated glucose tolerance or increased glucose clearance by Atg5. In addition, Atg5 Tg mice also showed enhanced insulin sensitivity following insulin stimulation for the ITT ( Fig. 3h ). Because insulin promotes hepatic triglyceride synthesis and the storage of triglyceride in white adipose tissue upon feeding and high levels of triglyceride may be associated with a shorter lifespan [24] , we measured triglyceride levels in the blood of Atg5 Tg mice. Compared with WT mice, triglyceride levels were slightly lower in young Atg5 Tg mice (4 months), but were evidently lower in old Atg5 Tg mice (18 months) ( Fig. 3i ). Furthermore, the levels of plasma leptin, an established regulator of body weight and energy balance [25] , were markedly decreased in young and old Atg5 Tg mice ( Fig. 3j ). These results show that Atg5 Tg mice exhibit improved metabolism, resulting in leanness. We also measured other ageing-associated parameters, such as the ratio of reduced glutathione to oxidized glutathione (GSH/GSSG) and mitochondrial oxygen consumption. Although the GSH/GSSG ratio, which represents the levels of intracellular antioxidants responsible for oxidative damage [26] , [27] , was decreased during ageing of both WT and Atg5 Tg mice in an age-dependent manner, its decrease was slow in the liver tissues of 12- and 24-month-old Atg5 Tg mice compared with WT mice ( Fig. 3k ). In addition, the oxygen consumption rate (OCR) was increased in the mitochondria of Atg5 Tg mice, as examined in mouse embryonic fibroblasts (MEFs) of passage number 2 ( Fig. 3l ). Compared with age-matched WT mice, Atg5 Tg mice showed significantly improved wire-hang endurance ( Fig. 3m ). It is likely that this represents a combination of changes in weight, lean/fat mass, motivation and muscle strength and so on. On the other hand, there was no difference in body temperature between the WT and Atg5 Tg mice ( Supplementary Fig. S4 ). When we assessed necropsy near the end of life using hematoxylin and eosin staining, we found normal age-dependent changes, including lipid accumulation in the liver, a cardiac fibrosis in the heart, and the loose contact of muscle fibres, that were more severe in 24-month-old WT mice than in age-matched Atg5 Tg mice ( Supplementary Fig. S5 ). These characteristics of the age-dependent changes are associated with the extended lifespan of Atg5 Tg mice. Atg5 Tg MEFs exhibit resistance to oxidative stress Because oxidative stress is considered as a prominent cause of ageing in mammals [26] , [27] , the observation that Atg5 Tg mice had higher levels of antioxidants than their littermates led us to investigate the oxidative stress response of cultured WT MEFs no. 1 and Atg5 Tg MEFs no. 6. When we directly assessed autophagy activity in primary cultured MEFs with western blotting, there were less p62 and more LC3 conversion in Atg5 Tg MEFs no. 6 than in WT MEFs no. 1 ( Fig. 4a,b,f ). Accordingly, treatment with rapamycin reduced the levels of p62 in Atg5 Tg MEFs no. 6 more evidently than in WT MEFs no. 1 ( Fig. 4b ). When MEFs were exposed to H 2 O 2 , Atg5 Tg MEFs no. 6 showed a greater resistance to cell death triggered by H 2 O 2 than WT MEFs no. 1 ( Fig. 4c,d ). In fact, only 15% of Atg5 Tg MEFs were dead at 24 h after treatment with H 2 O 2 , compared with 80% of WT MEFs ( Fig. 4c,d,e ). Treatment with 3-methyladenine (3-MA), an autophagy inhibitor [28] , accelerated H 2 O 2 -induced cell death in WT and Atg5 Tg MEFs ( Fig. 4d ). Consistently, treatment with bafilomycin A1 (Baf.A1), a potent and specific inhibitor of vacuolar H + ATPase in lysosomes and, thus, of autophagy [29] , sensitized Atg5 Tg MEFs to H 2 O 2 (15 to 40%), and this sensitizing effect was more profound in Atg5 Tg MEFs than in WT MEFs (80 to 90%). In addition, western blot analysis showed that the levels of LC3 II were higher in Atg5 Tg MEFs than in WT MEFs when exposed to H 2 O 2 ( Fig. 4f ). On the other hand, WT and Atg5 Tg MEFs showed similar susceptibilities to cell death triggered by other death signals, for example, etoposide, staurosporine and TNF-α/cycloheximide ( Supplementary Fig. S6 ). 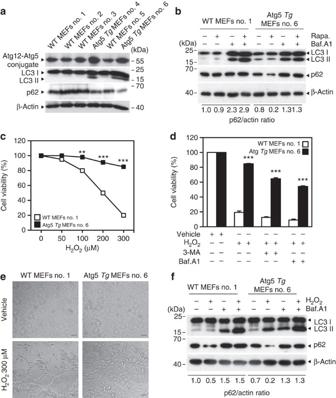Figure 4: Tolerance of Atg5TgMEFs to oxidative stress via autophagy activity. (a) Comparison of Atg12-Atg5 conjugate levels in WT and Atg5TgMEFs by western blot analysis. MEFs from WT and Atg5Tgmice were cultured at embryonic day 13, after which cell extracts were examined by western blot analysis using anti-Atg5 and anti-β-actin antibodies. (b) Increased conversion of LC3 and reduced expression of p62 in Atg5TgMEFs no. 6 by rapamycin and/or Baf.A1. WT MEFs no. 1 and Atg5TgMEFs no. 6 in passage number 3 were incubated for 48 h with 10 μM rapamycin in the absence or presence of Baf.A1, and cell extracts were then analysed by western blotting. The signals on the blot were quantified by densitometric analysis and represented as the ratio of p62 to β-actin. (c,d) Increased resistance of Atg5TgMEFs to oxidative stress. WT MEFs no. 1 and Atg5TgMEFs no. 6 were treated for 24 h with 50, 100, 200 and 300 μM H2O2(c) or 300 μM H2O2in the absence or presence of 5 mM 3-MA or 20 nM Baf.A1 (Baf.A1) (d). Cell viability was assessed by propidium iodide staining. The values are the mean±s.e.m. (n=3). **P<0.001, ***P<0.0001 versus control; Student’st-test. (e) Representative photographs showing the resistance of Atg5TgMEFs to oxidative stress. Primary cultured WT and Atg5TgMEFs were treated with 300 μM H2O2for 24 h and then observed under a light microscope. Scale bars, 50 μm. (f) Effect of oxidative stress on the autophagy activity in Atg5TgMEFs. WT MEFs no. 1 and Atg5TgMEFs no. 6 were treated with 100 μM H2O2for 24 h in the presence or absence of 20 nM Baf.A1, and cell extracts were analysed by western blotting. About 10 and 30 μg of proteins were used for LC3 (upper panel) and p62 (bottom panel) detection, respectively. β-Actin served as a control. Figure 4: Tolerance of Atg5 Tg MEFs to oxidative stress via autophagy activity. ( a ) Comparison of Atg12-Atg5 conjugate levels in WT and Atg5 Tg MEFs by western blot analysis. MEFs from WT and Atg5 Tg mice were cultured at embryonic day 13, after which cell extracts were examined by western blot analysis using anti-Atg5 and anti-β-actin antibodies. ( b ) Increased conversion of LC3 and reduced expression of p62 in Atg5 Tg MEFs no. 6 by rapamycin and/or Baf.A1. WT MEFs no. 1 and Atg5 Tg MEFs no. 6 in passage number 3 were incubated for 48 h with 10 μM rapamycin in the absence or presence of Baf.A1, and cell extracts were then analysed by western blotting. The signals on the blot were quantified by densitometric analysis and represented as the ratio of p62 to β-actin. ( c , d ) Increased resistance of Atg5 Tg MEFs to oxidative stress. WT MEFs no. 1 and Atg5 Tg MEFs no. 6 were treated for 24 h with 50, 100, 200 and 300 μM H 2 O 2 ( c ) or 300 μM H 2 O 2 in the absence or presence of 5 mM 3-MA or 20 nM Baf.A1 (Baf.A1) ( d ). Cell viability was assessed by propidium iodide staining. The values are the mean±s.e.m. ( n =3). ** P <0.001, *** P <0.0001 versus control; Student’s t -test. ( e ) Representative photographs showing the resistance of Atg5 Tg MEFs to oxidative stress. Primary cultured WT and Atg5 Tg MEFs were treated with 300 μM H 2 O 2 for 24 h and then observed under a light microscope. Scale bars, 50 μm. ( f ) Effect of oxidative stress on the autophagy activity in Atg5 Tg MEFs. WT MEFs no. 1 and Atg5 Tg MEFs no. 6 were treated with 100 μM H 2 O 2 for 24 h in the presence or absence of 20 nM Baf.A1, and cell extracts were analysed by western blotting. About 10 and 30 μg of proteins were used for LC3 (upper panel) and p62 (bottom panel) detection, respectively. β-Actin served as a control. Full size image Furthermore, protein oxidation, which is usually detected in aged tissues and can serve as a marker associated with ageing [30] , [31] , was enhanced in the murine liver following a tail vein injection of siRNA-Atg5 and thus showing reduced Atg5 expression ( Supplementary Fig. S7a ). On the other hand, an enzyme-linked immunosorbent assay showed that the levels of oxidized proteins were reduced in Atg5 Tg MEFs no. 6, compared with WT MEFs no. 1 ( Supplementary Fig. S7b ). Interestingly, this reduction in Atg5 Tg MEFs no. 6 was abolished by the treatment with 3-MA; the levels of oxidized proteins equally increased in both WT MEFs no. 1 and Atg5 Tg MEFs no. 6. Thus, it appears that the enhanced autophagy seen in Atg5 Tg MEFs is crucial for their tolerance to protein oxidation and oxidative stress-induced cell death. In summary, Atg5 Tg mice exhibited an extended lifespan and lean phenotype, which might be attributed to enhanced autophagy activity via the regulation of oxidative stress and ageing-associate metabolism, such as insulin sensitivity. Over the years, the hypothesis that autophagy is involved in ageing has been largely studied using cell culture and model organisms. The accumulation of damaged macromolecules and organelles during ageing occurs due to reduced autophagy activity [19] , [32] , [33] . Thus, the inactivation of autophagy by the knockdown of Atg1, beclin 1, Atg7, LC3, Atg9 and Atg12 leads to reduced lifespan as a result of the premature onset of ageing-related symptom in model organisms [34] . Indeed, most studies on autophagy in ageing have been carried out in model organisms, such as yeast, C. elegans and D. melanogaster , using loss-of-function mutants of Atg genes and caloric restriction models [35] , [36] . On the other hand, knockout mice of Atg3 (ref. 37 ), Atg5 (ref. 15 ), beclin 1 (refs 38 , 39 ), Atg7 (ref. 40 ), Atg9 (ref. 41 ), Atg16L (ref. 42 ) and FIP200 (ref. 43 ) were embryonic or neonatal lethal, which made it impossible to examine the role of autophagy in mammalian longevity. Some reports indicating that the constitutive loss of Atg genes in the central nervous system of mice causes neurodegeneration and a shortened lifespan partly illustrate the tissue-specific role of autophagy in mammalian longevity [15] , [40] . In addition, studies showing that FoxO [44] , p53 (ref. 45 ) and SIRT1 (ref. 46 ) regulate lifespan and autophagy activity are interesting, but are insufficient to support a role of increased autophagy as well as autophagy regulation in enhanced longevity because they are multi-function proteins. Similarly, a recent report that treatment with rapamycin increases lifespan in mice [13] could, in part, reflect the fact that the activation of autophagy may contribute to longevity in mammals. However, this perspective also becomes more complicated by the observation that deletion of ribosomal S6 protein kinase 1, a component of the nutrient-responsive mTOR-signalling pathway, also affects lifespan in mice [47] . Unlike the aforementioned reports, the present study used gain-of-function Atg5 Tg mice to demonstrate a role of autophagy activation in the extension of mammalian lifespan. We explored a role of autophagy in lifespan using Atg5 Tg mice. Among the Atg genes, Atg5 has critical role in autophagy activation by participating in two essential pathways, that is, Atg12-Atg5 conjugation and LC3 lipidation. As far as the hypothesis that Atg5 overexpression alone is able to enhance autophagy activity is concerned, we have clearly and consistently observed a significant increase of autophagy activity in Atg5 Tg mice, as measured by the number of autophagosomes under an electron microscope, LC3 II conversion and p62 accumulation and the fluorescence intensity of GFP-LC3 in Atg5 Tg /GFP-LC3 double Tg mice. In parallel, we and other groups also observed that overexpression of Atg genes in mammalian cells increases autophagy [48] , [49] . Although overactivation of excessive autophagy may not always be beneficial, we believe that the ectopic expression of Atg5 in these mice regulates autophagy flux. Mice deficient for Atg5 appear almost normal at birth, but die within 1 day due to a suckling defect [15] . Conversely, Atg5 Tg mice were normal at birth, but showed leanness with loss of weight during ageing despite having the same food intake as their WT littermates. Many studies on long-lived mice imply a critical role of insulin in longevity and suggest that leanness is closely linked to a metabolic condition that favours longevity through the regulation of insulin signalling [50] , [51] , [52] . In addition, the inactivation of autophagy by the knockdown of beclin 1, Atg 7 or Atg 12 shortens the lifespan of daf-2 mutant worms [6] , [7] , [8] , [9] , [10] . All of these reports suggest that autophagy may regulate ageing through the conserved insulin/IGF-1 signalling pathway. As we also observed insulin and glucose tolerance in Atg5 Tg mice, the regulation of insulin signalling may contribute to the leanness of these mice [53] . Glutathione is a ubiquitous cellular constituent that is the most abundant thiol-reducing agent in mammalian tissues and its levels are usually decreased when cells or mice age [54] . Our observation that the concentration of glutathione remains higher over time in Atg5 Tg mice than in WT mice implies that enhancing autophagy activity may also affect oxidative stress. Consistently, cultured Atg5 Tg MEFs were tolerant to oxidative stress and protein oxidation in an autophagy activity-dependent manner. These data suggest that the observed tolerance to oxidative stress may contribute to the extended lifespan of Atg5 Tg mice. In addition, the improved performance of Atg5 Tg mice in the wire-hang test demonstrates the enhanced physical activity, including motor activity and strength. Bearing in mind that increased fluorescence was evident in the muscles of Atg5/GFP-LC3 Tg mice, the enhanced motor function of Atg5 Tg mice might be attributed to enhanced autophagy driven by Atg5. Accordingly, enhanced oxygen consumption in Atg5 Tg MEFs may be in a line with this enhanced physical activity of Atg5 Tg mice. Collectively, we attribute the improved insulin sensitivity and reduced oxidative stress to enhanced autophagy. Although it still remains to be seen as to how autophagy regulates those signals in detail, we propose that enhanced autophagy in Atg5 Tg mice has a crucial role in the extension of mammalian lifespan with leanness. Reagents Antibodies, cell culture reagents and their sources were as follows: anti-LC3, anti-Atg5 and anti-p62 (polyclonal; Novus Bio., Littleton, USA); anti-β-actin (Cell Signaling Technology, Danvers, MA, USA); DMEM (WelGENE, Daegu, Korea); and foetal bovine serum (FBS) (Invitrogen, Houston, TX, USA). All other biochemicals used were of the highest purity available and were obtained from regular commercial sources. Generation of Atg5 transgenic mice A full-length untagged cDNA encoding rodent Atg5 was subcloned into Sal I site of p CAGGS vector [20] , which contains the cytomegalovirus enhancer, the chicken β-actin promoter and a rabbit β-globin poly (A). The resulting plasmid, p CAGGS- Atg5 , was digested using Sal I and Xho I to isolate the transgenic cassette. The isolated cassette was injected into C57BL/6 mouse embryos and the mouse embryos (fertilized one-cell zygotes) were then implanted into female mice (Macrogen Inc., Seoul, Korea). Atg5 Tg mice were identified by genomic DNA PCR analysis using genomic DNA prepared from their tails. Positive F0 mice were identified using a synthetic oligonucleotide (forward, 5′-CGG CTC TAG AGC CTC TGC TAA C-3′) corresponding to the p CAGGS and an oligonucleotide (reverse, 5′-TGA TGG CCC AAA ACT GGT-3′) from the Atg5 cDNA. Four independent founder lines were identified and mated to C57BL/6 mice. All mice were maintained under a 12:12 h light:dark cycle with access to food and water ad libitum. All animal protocols were approved by the Gwangju Institute of Science and Technology and Seoul National University Standing Committees on Animals. Mouse longevity study Mice were housed in groups of four to eight same-sex littermates under specific pathogen-free conditions. Individuals were monitored daily and weighed monthly, but were otherwise left undisturbed until they died. Survival was assessed using male and female mice, and all animals were dead by the time of this report. Kaplan–Meier survival curves were constructed using known birth and death dates, and differences between groups were evaluated using the log-rank test. Y-maze test was performed using the previously established methods [55] . Electron microscopy analysis Freshly isolated white adipose tissue from mice were fixed with 2.5% glutaraldehyde/4% paraformaldehyde in 0.1 M cacodylate buffer for 2 h. The samples were processed and thin sections (90 nm) were cut on a Reichert Ultracut E microtome. Sections were viewed at 80 kV with a JEOL 1200EX transmission electron microscope. Micrographs were taken in the Philips CM12 (15–20 per sample) by random sampling with magnification form × 3,000–20,000. Autophagic vacuoles were counted and measured in 50 random cells, averaged and expressed as the number of autophagic vacuoles per cell. Delivery of siRNA into mice Atg5 Tg mice (8-week old) were injected with siRNA-Atg5 (1 mg kg −1 ) or Atg5-HA (0.5 mg kg −1 ) via tail vein, and 48 h later, liver extracts were analysed by western blotting [56] . Determination of body weight and food intake Body weight and food intake of mice were recorded and measured weekly. To estimate food consumption, food intake was assessed by weighing the food in each cage dispenser, including the food that was spilled on the floor of the cage. Blood and plasma measurement Blood tests were performed with kits following the manufacturer’s instruction; glucose with One Touch Ultra Smart blood glucose monitoring system (Johnson & Johnson); Mouse TG with kit from Life Sciences Advanced Technologies. For plasma measurement, blood samples were collected from mice tail with heparinized microhematocrit capillary tubes (Fisher) and plasma was obtained by centrifugation of the blood samples for 3 min. Leptin level was measured by ultra sensitive mouse leptin ELISA kit (Biovendor Lab. Inc.). GTT and ITT For GTT, mice were starved overnight and intraperitoneal (i.p.) injected with 20% glucose at a dose of 2 g kg −1 body weight. Blood was obtained from the tail at time points 0, 15, 30, 60, 90 and 120 min for glucose measurement. For ITT, mice were starved for 6 h and i.p. injected with 0.75 U recombinant human insulin per kg body weight (Sigma). Blood was obtained from the tail at the time points for glucose measurement. Measurements of OCR OCR of MEFs was measured in a Seahorse Bioscience XF24 Extracellular Flux Analyzer (North Billerica, MA, USA). In XF24-well microplates (Seahorse Bioscience), MEFs were seeded with 4 × 10 4 cells per well in DMEM containing 10% FBS, and for the XF24 assay, cells were placed in the instrument and basal oxygen consumption was recorded in three times. The proton leak rate was determined by the subsequent addition of oligomycin (4 μg ml −1 ). At the end of the run, 1 μM rotenone was added to determine the mitochondria-independent oxygen consumption. Protein concentration in each well was determined with the bicinchoninic acid method in cell lysates. Cellular assays MEFs were prepared as previously described [20] . Briefly, mouse embryonic tissue from WT and Atg5 Tg mice (E13.5) was minced with a razor blade, trypsinized at 37 °C for 5 min and then incubated with DMEM supplemented with 10% FBS. MEFs were frozen for further use. Determination of glutathione content GSH/GSSG contents were measured using the luminescence-based system (Promega) in tissue and cultured cells. Muscular strength Muscular strength was tested at 2-, 6- and 12-month-old age with the wire-hang tests. The mouse was trained to perform rid-hanging exercise for 15 days and then placed on a horizontal wire mesh that was then inverted and waved gently, so that the mouse gripped the wire. The time that each mouse remained on the wire was recorded. Three trials were performed for each mouse for three consecutive days, and the average was used for statistical analysis. Western blot analysis Tissue samples were homogenized in lysis buffer (2 mM DTT, 10% glycerol, 1% Triton X-100, 2 mM 1,2-diaminocyclohexane-N,N,N′,N′-tetraacetic acid and 25 mM Tris–HCl, pH 7.8), after which protein levels were determined using the method of Bradford (Bio-Rad). Samples of cell extract containing 3–5 μg of proteins in a buffer (60 mM Tris–HCl, pH 6.8, 1% SDS, 10% glycerol and 0.5% β-mercaptoethanol) were subjected to SDS–polyacrylamide gel electrophoresis and then transferred to nitrocellulose membranes using a Semi-Dry Transfer System (Bio-Rad). The membranes were blocked with TBST buffer (20 mM Tris–Cl, pH 7.5, 150 mM NaCl and 0.2% Tween 20) containing 3% bovine serum albumin, proved with primary and secondary antibodies, and proteins were visualized using enhanced chemiluminescence. Analysis of protein carbonyls and oxidation Oxidatively modified proteins in the liver and MEFs were analysed by Western blot analysis using anti-DNP antibody (1:100 dilution) [57] . Statistical analyses All statistical analyses were performed using SigmaStat 10.0 software. Data were compared using two-tailed Student's t -tests or one-way analysis of variance. How to cite this article: Pyo, J.-O. et al. Overexpression of Atg5 in mice activates autophagy and extends lifespan. Nat. Commun. 4:2300 doi: 10.1038/ncomms3300 (2013).